Upright human gait did not provide a major mechanical challenge for our ancestors Habitual bipedalism is considered as a major breakthrough in human evolution and is the defining feature of hominins. Upright posture is presumably less stable than quadrupedal posture, but when using external support, for example, toddlers assisted by their parents, postural stability becomes less critical. In this study, we show that humans seem to mimic such external support by creating a virtual pivot point (VPP) above their centre of mass. A highly reduced conceptual walking model based on this assumption reveals that such virtual support is sufficient for achieving and maintaining postural stability. The VPP is experimentally observed in walking humans and dogs and in running chickens, suggesting that it might be a convenient emergent behaviour of gait mechanics and not an intentional locomotion behaviour. Hence, it is likely that even the first hominis may have already applied the VPP, a mechanism that would have facilitated the development of habitual bipedalism. Habitual terrestrial bipedalism has often been considered the evolutionary event that separated humans from apes [1] , [2] . Because bipedalism enhances the ability to gather small fruit from short trees and frees the hands for tool use, bipedalism might have not only been an adaptation to an ecological niche but also a prerequisite for cultural development and for the evolution of modern humans [3] , [4] . However, an important selection criterion in evolution is the efficiency of gait [1] , [5] ; an efficient bipedal gait requires straightened legs and an upright trunk as opposed to 'bent-hip-bent-knee walking' [6] . Early habitual bipeds such as Australopithecus afarensis and perhaps even Ardipithecus ramidus ('Ardi') presumably already used an upright gait [7] , [8] , [9] , [10] . Walking upright entails advantages but also raises new challenges including load distribution on two legs only and stabilization of the upright posture. Although the increased load per leg can be compensated by extended legs [4] , the intuitively expected instability of bipedal gait seems to be a rather complex challenge. The dramatically reduced area of support compared with quadrupedal walking and an elevated centre of mass (CoM) in upright bipedal gait provide reason to assume increased instability. The system resembles an inverted pendulum that easily falls over when perturbed. However, this relation is only valid for static scenarios. In human walking, the point of application of the ground reaction force (GRF) moves with respect to the CoM throughout a walking cycle ( Fig. 1a ). This fundamental difference compared with an inverted pendulum ( Fig. 1b ) is the basis for a stabilization mechanism that does not rely on the instantaneous area of support. 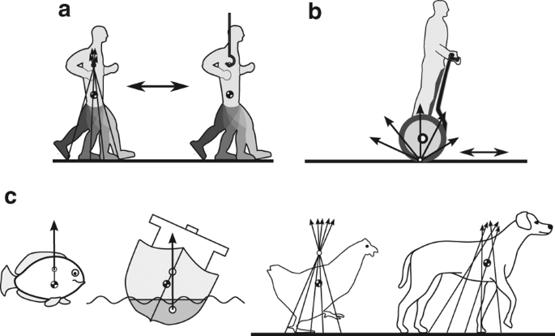Figure 1: The virtual pendulum (VP) concept. (a) A physical pendulum is mimicked when the ground reaction forces (GRFs) intersect above the centre of mass (CoM). Such systems are termed VPs. This behaviour is found in human walking (cf.Fig. 3) and is in contrast to a feedback-stabilized inverted pendulum (b). Whereas inathe origin of force moves with respect to the body, in the inverted pendulum shown inbthe direction of the force is adjusted to maintain the upright posture. Hence, inb, the postural stability is achieved by appropriate acceleration, whereas in VP systems the coupling of posture to motion can be much weaker (see text). (c) A VP is found in different systems, for example, in fish and ships, in which the GRF is replaced by the buoyancy force, or in other animals such as walking dogs and running chickens (see alsoFig. 3). A single intersection point is not necessary for a VP system and cannot always be found (seeFig. 3and text). Figure 1: The virtual pendulum (VP) concept. ( a ) A physical pendulum is mimicked when the ground reaction forces (GRFs) intersect above the centre of mass (CoM). Such systems are termed VPs. This behaviour is found in human walking (cf. Fig. 3 ) and is in contrast to a feedback-stabilized inverted pendulum ( b ). Whereas in a the origin of force moves with respect to the body, in the inverted pendulum shown in b the direction of the force is adjusted to maintain the upright posture. Hence, in b , the postural stability is achieved by appropriate acceleration, whereas in VP systems the coupling of posture to motion can be much weaker (see text). ( c ) A VP is found in different systems, for example, in fish and ships, in which the GRF is replaced by the buoyancy force, or in other animals such as walking dogs and running chickens (see also Fig. 3 ). A single intersection point is not necessary for a VP system and cannot always be found (see Fig. 3 and text). Full size image Assuming that the body would be supported above the CoM, such as when walking with crutches or brachiating in trees, the inverted pendulum could be transformed into a regular physical pendulum. Perturbations could then be tolerated because they would result in pendulum-like swinging motions, allowing the system to react adequately if necessary. Appropriate support can also be mimicked inherently by the system by redirecting the GRF to a point above the CoM. Small perturbations would automatically lead to torques restoring posture similar to the function of a physical pendulum ( Fig. 1a ). The concept of mimicking a physical pendulum can be found in different contexts ( Fig. 1c ) and is here termed the virtual pendulum (VP) concept. Turning an inverted pendulum into a VP differs from the approach of using postural feedback for explaining dynamic stability during bipedal gait. The VP approach does not include sensory feedback on the current posture (body pitch). In contrast to a feedback-stabilized inverted pendulum, as displayed in Figure 1b, in which acting forces intersect below the CoM at the contact point with the ground, forces intersect above the CoM in VP systems. A moving point of origin of force with respect to the body, as typical for legged locomotion, is an important prerequisite for a VP. In human walking, a force intersection point clearly above the CoM can be observed, indicating the realization of the VP concept. Here, the VP concept is represented by one single point, which is termed the virtual pivot point (VPP). In this paper, we demonstrate how the VP concept explains dynamic stability during upright bipedal gait and provide experimental evidence that this concept is not exclusive to human walking. Further, we discuss the importance of this concept in the development of upright human walking. Model In biomechanics, conceptual models are widely used to elucidate specific aspects of bipedal gait. The simplest walking model consists of a point mass on rigid legs [11] and predicts walking and running to be optimal modes of locomotion [12] . Despite the explanatory power of the model for many aspects [13] , [14] , [15] , the lack of compliance in the legs does not allow this model to predict typical experimental GRF patterns that can be considered as the fingerprint of a gait. Human-like GRF patterns are generated by the bipedal spring-mass model [16] , [17] , [18] , [19] , in which the rigid legs of the simplest model are replaced by springs. Here, we follow the tradition of conceptual models and extend this model by replacing the point mass of the original model with a rigid body, thereby moving the CoM above the hip as is the case in humans ( Fig. 2a ). The body essentially represents an unstable inverted pendulum that needs to be stabilized on top of two legs. Stability is implemented using the VP concept. 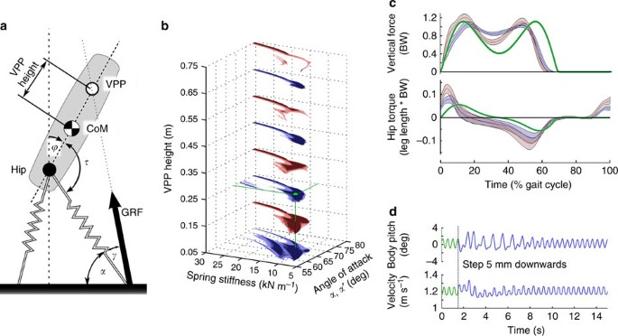Figure 2: Results of the VPP model. (a) The VPP model consists of a rigid body above two massless leg springs. A hip torque is introduced to redirect the GRF to the VPP located above the CoM. (b) This graph shows parameter configurations for which the model reached at least 10 steps (light areas), 25 steps (medium areas) or 50 steps (dark areas) from non-steady state (seeMethodssection. An animation of the model falling down after several successful steps is available inSupplementary Movie 2). The simulation was stopped after 50 steps. For a motivation of this steps-to-fall method, see Seyfarthet al.19In red areas, the leg is aligned with respect to the ground (angle of attackα), whereas in blue areas the leg is aligned with respect to the body (angle of attackα′, whereα=α′+ϕ). For visual presentation, areas are drawn every 10 cm. The configuration at the location shown in green (spring stiffness: 13 kN m−1,α′=69°, VPP height=0.25 m) was used for calculation shown incandd. (c) The model generated hip torque and GRF patterns that resemble those of human walking (BW, bodyweight). The solid green lines depict simulation results, and the blue and red areas correspond to the mean and standard deviation of our experimental data at 1.1 and 1.6 ms−1, respectively. (d) Starting from a periodic solution (green region), a small disturbance of a 5 mm step is negotiated by the model without any parameter adaptation, indicating that the VP concept provides basic postural stability. Here, the model shows partially35stable solutions, that is, after a small perturbation, the model generally approaches another solution. A hip torque during the stance of each leg is introduced to redirect its GRF to a VPP somewhere along the body's long axis, as shown in Figure 2a . Figure 2: Results of the VPP model. ( a ) The VPP model consists of a rigid body above two massless leg springs. A hip torque is introduced to redirect the GRF to the VPP located above the CoM. ( b ) This graph shows parameter configurations for which the model reached at least 10 steps (light areas), 25 steps (medium areas) or 50 steps (dark areas) from non-steady state (see Methods section. An animation of the model falling down after several successful steps is available in Supplementary Movie 2 ). The simulation was stopped after 50 steps. For a motivation of this steps-to-fall method, see Seyfarth et al . [19] In red areas, the leg is aligned with respect to the ground (angle of attack α ), whereas in blue areas the leg is aligned with respect to the body (angle of attack α ′, where α = α ′+ ϕ ). For visual presentation, areas are drawn every 10 cm. The configuration at the location shown in green (spring stiffness: 13 kN m −1 , α ′=69°, VPP height=0.25 m) was used for calculation shown in c and d . ( c ) The model generated hip torque and GRF patterns that resemble those of human walking (BW, bodyweight). The solid green lines depict simulation results, and the blue and red areas correspond to the mean and standard deviation of our experimental data at 1.1 and 1.6 ms −1 , respectively. ( d ) Starting from a periodic solution (green region), a small disturbance of a 5 mm step is negotiated by the model without any parameter adaptation, indicating that the VP concept provides basic postural stability. Here, the model shows partially [35] stable solutions, that is, after a small perturbation, the model generally approaches another solution. Full size image Simulations The model generated walking solutions similar to those of the underlying spring-mass template, which can adjust to subtle changes in the ground level ( Fig. 2d ). Animations of successful disturbance rejection, as well as an improper model configuration that fails after several steps, are available in Supplementary Movies 1 and 2 . Even though no damping was introduced, body pitch oscillation after perturbation diminished over time, which is different from the behaviour of a physical pendulum. In this model, stability of the underlying gait model seems to affect postural sway. Replacing the point mass of the template by a trunk offers a new reference frame given by the body's long axis, which can be used to align the leg in preparation of touch down. Hence, body-specific sensory signals instead of global information (for example, gravity direction) can be used for leg placement. The results of our simulation showed that this feature may not only preserve but even increase the stability of the model ( Fig. 2b ). In the model, a second functional role of the trunk lies in the adjustment of speed during locomotion: Because the GRF is always directed to the VPP, the forward and backward lean of the trunk must be accompanied by the acceleration and deceleration of the system, respectively. Thus, adjusting the VPP location offers a simple way to change the speed of the model. With respect to model performance, adding a trunk to the model seems to be a greater chance than challenge when the VP concept is applied. Despite its simplicity, the VPP model is capable of predicting hip torque patterns similar to those observed in human walking ( Fig. 2c ). In this model, the similarity is lost when replacing the VP scheme by a pitch-proportional hip torque control scheme using a global reference frame. However, the loss of similarity by direct feedback on the posture is not lost in all cases, as shown, for instance, by the model of Geyer and Herr [20] . When applying the VP concept, the GRF remains aligned towards the body until the leg spring is unloaded, which is required to achieve steady ground contacts. With these mechanically attractive and biologically reasonable properties, the VP concept seems to be suitable for describing human gait and may be used as a basis for more detailed models of human locomotion. VPP location In experimental studies, the VPP for each step can be defined as the single point at which (i) the total transferred angular momentum remains constant and (ii) the sum-of-squares difference to the original angular momentum over time is minimal, if the GRF is applied at exactly this point. For human walking, the correspondingly calculated VPP is located 5–70 cm above the CoM ( Fig. 3a,b ). A similar range of VPP location is also predicted by the model, in which most stable solutions can be found for VPP heights of approximately 1–50 cm ( Fig. 2b ). If VPP height reaches the boundary of this range, only few gait patterns remain stable. For a given VPP location, the model is stable for a range of different leg stiffness and angles of attack ( Fig. 2d ). The results of the model showed that hip torque magnitude and VPP location are tightly related. Thus, experimentally measured VPP location may be a sensitive measure to assess human gait in general and during development and in health and disease. 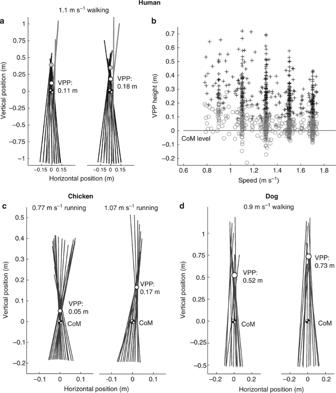Figure 3: The VPP in experimental data. (a) Two subsequent steps typical for human walking are shown. Here, the coordinate system originates at and moves with the CoM. Lines show the total ground reaction force at different times, originating at the centre of pressure and pointing along the line of action of the force. The ground reaction forces are clearly focused above the CoM. The white circle shows the calculated effective VPP (see text). If the impact force around touchdown (grey lines) is omitted, a very clear intersection point would occur (here, grey circles at 0.39 and 0.35 m, respectively). The impact can then be regarded as disturbance to the system. (b) Calculated VPP positions from six subjects walking on an instrumented treadmill at different speeds are shown. Grey circles show calculated VPP heights with impact forces, black crosses show VPP heights without impact forces. (c) In running chickens, a clear VPP was observed. In our data, VPP height is strongly coupled to running speed. (d) Although less focused than in running chickens or walking humans, walking dogs also show a VPP. Figure 3: The VPP in experimental data. ( a ) Two subsequent steps typical for human walking are shown. Here, the coordinate system originates at and moves with the CoM. Lines show the total ground reaction force at different times, originating at the centre of pressure and pointing along the line of action of the force. The ground reaction forces are clearly focused above the CoM. The white circle shows the calculated effective VPP (see text). If the impact force around touchdown (grey lines) is omitted, a very clear intersection point would occur (here, grey circles at 0.39 and 0.35 m, respectively). The impact can then be regarded as disturbance to the system. ( b ) Calculated VPP positions from six subjects walking on an instrumented treadmill at different speeds are shown. Grey circles show calculated VPP heights with impact forces, black crosses show VPP heights without impact forces. ( c ) In running chickens, a clear VPP was observed. In our data, VPP height is strongly coupled to running speed. ( d ) Although less focused than in running chickens or walking humans, walking dogs also show a VPP. Full size image Stabilizing posture by applying the VP concept is not unique to human walking. Similar observations have been made in other animals, including in dogs when walking on a treadmill ( Fig. 3d ) and in chickens when walking and running over the ground ( Fig. 3c ). Similar to the spring-mass model, the VP concept describes a mechanical behaviour rather than an explicit movement trajectory. The VP concept combined with the spring-mass model can tolerate small disturbances and compensates for such disturbances by its inherent mechanical properties without the need for active regulation. This observation is a possible explanation of why natural walking feels effortless. For each model, there is a trade-off between its simplicity and its limitations. This model was limited to the parasagittal plane, and additional stability challenges originating from three-dimensional motion were neglected. In addition, the model did not contain a foot, and the trunk, arms, head and leg masses were combined in a rigid trunk. These additional aspects can be modelled using different modelling approaches [20] , [21] , [22] , [23] that are often linked to the basic models. However, in this study, we followed the tradition of conceptual models focussing on the point of interest. The existence of a VP in different animals suggests that the VP might be the result of mechanical circumstances rather than being a primarily intended locomotion pattern. In the following, this theory is discussed using the example of bipedal human walking. For a VPP in human walking, torques extending the hip are required in the first part of the stance, and torques flexing the hip are required in the last part of the stance. These torques reduce the horizontal forces. Further, these torques generate leg retraction and protraction as required at the time of transition between contact and swing. Hip extension torques before ground contact, as observed in experimental data ( Fig. 2c ), retract the leg and hence prepare the leg for ground contact. Apparently, the hip torques required for leg protraction and retraction during steady locomotion also provide the VP and facilitate postural stability. Thus, using the VP concept requires almost no additional effort. The VP concept can be considered a general template [24] for locomotion, similar to the spring-like leg behaviour found in various animals [18] , [25] , [26] . Nature seems to take advantage of the attractive properties of mechanical templates that facilitate stable gait without the need for precise trajectory planning [16] , [19] . Jointly implemented as the VPP model, these two templates combined are able to describe upright human walking. Moreover, the supportive function of the VP may have assisted the erection of hominine walking. Recent research suggests that humans did not evolve from a knuckle-walking ancestor [27] . Instead, the erection of locomotion likely took place in an arboreal environment, similar to the environment in which orangutans live even at present. When brachiating through trees, straighter legs and a more upright posture can be observed as an adaptation to more flexible branches [28] , making the gait kinematically more similar to modern human walking. This theory is supported by observations of fossils of the recently presented early hominine A. Ramidus 'Ardi', who seems to have retained arboreal locomotion capabilities but did not rely on physical suspension [29] . On the basis of (i) the presence of a VPP in various animal and human gaits, (ii) the illustrated mechanism that facilitates the VPP in human walking and (iii) the presumed similarity of ancestral and modern human gait [28] , it can be concluded that 'Ardi' may have overcome the apparent instability of upright gait by using the VP concept. If this theory holds true, instability was likely not an obstacle in the evolution of human bipedalism. Modelling The model's equations of motion are with mass m =80 kg and moment of inertia J =5 kg m −2 . r VPP denotes VPP height, F x and F y denote the horizontal and vertical GRF, respectively. GRF is the sum of leg spring force F S pointing along the leg axis and force F τ induced by the hip torque and acting perpendicular to the massless leg spring. The magnitude of F S is given by F S = k ( L 0 − L ), with k denoting spring stiffness and L 0 and L denoting spring rest length and current length, respectively. The magnitude of F τ is F τ = F S tan( γ ). Here, positive values of F τ correspond to a clockwise rotation of F S . The corresponding hip torque τ is calculated by τ = L · F S tan( γ ). The initial conditions for Figure 2b were Initial height was calculated such that the energy stored in the spring equalled 3J. The remaining energy from a total of 900 J was used for motion in walking direction. The model was implemented in Matlab R2009a using the Simulink 7 toolbox (Mathworks). Experimental data To compare hip torques predicted by the VPP model with hip torques observed in human gait, previously collected data for 21 healthy subjects walking and running on a treadmill were analysed [30] . Inverse dynamics were calculated by a sequential algorithm, taking soft tissue dynamics into account [31] . Calculated hip torques were normalized to each subject's body weight, leg length and gait cycle, and then averaged to give an overall mean including all steps of all subjects. CoM motion was obtained by integrating the GRFs twice. Initial values for velocity were estimated from kinematic measurements. For human walking, the height of the sacrum was taken as initial CoM height [32] . For dogs and chickens, initial CoM heights were estimated according to literature [33] , [34] . How to cite this article: Maus, H.-M. et al . Upright human gait did not provide a major mechanical challenge for our ancestors. Nat. Commun. 1:70 doi: 10.1038/ncomms1073 (2010).